Linkage of genetic drivers and strain-specific germline variants confound mouse cancer genome analyses 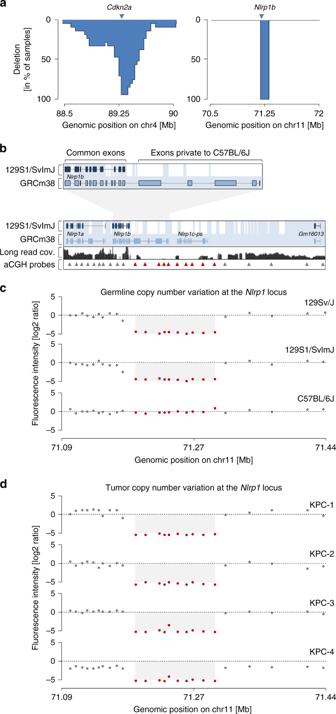Fig. 1: Strain-specific haplotype variation at theNlrp1locus in 129S and C57BL/6J mice. aOverlay of homozygous somatic deletions at the “classic” tumor suppressor locusCdkn2ais shown (n= 21 KC mice; for each tumor the homozygously deleted region is shown; data from ref.13). For comparison, overlay of copy number alterations in primary pancreatic cancer cell cultures withNlrp1locus deletions, as detected by aCGH (exemplary KPC mice are shown,n= 4; see also details of individual tumors in Fig. 1d).Yaxis, frequency of genomic regions homozygously deleted in the cohort.bStrain-specific haplotype diversity at the mouseNlrp1locus on chr11. Genomic alignment of theNlrp1129S1/SvImJlocus toNlrp1C57BL/6J(GRCm38 mouse reference genome). Sequence homology of C57BL/6J and 129S1/SvImJ is highlighted in light blue. Genomic regions without homology in 129S1/SvImJ are depicted in white (data adapted from ref.5). Upper panel: zoom-in ofNlrp1b(exon/intron lengths not proportional to genomic distances). Lower panel, middle row: read coverage of theNlrp1C57BL/6Jlocus in a KPC mouse withTrp53ENG, as detected by nanopore long-read sequencing. Lower panel, bottom row: genomic position of oligonucleotide probes of the Agilent SurePrint G3 Mouse CGH 240 K array. Red arrowheads, aCGH probes located within theNlrp1locus alteration described by Niknafs et al.1(compare to Fig. 1c, d).cGermline CNV profiles at theNlrp1locus in three inbred mouse strains. DNA from indicated strains was hybridized against DNA from C57BL/6J. Red dots, aCGH probes within theNlrp1locus alteration (data from ref.6).dRecurrentNlrp1locus alterations in primary pancreatic cancer cell cultures with identical genomic boundaries (exemplary KPC mice are shown). The Agilent SurePrint G3 Mouse CGH 240 K array was used similar to Niknafs et al.1and Fig. 1c. Red dots, aCGH probes within theNlrp1locus alteration. 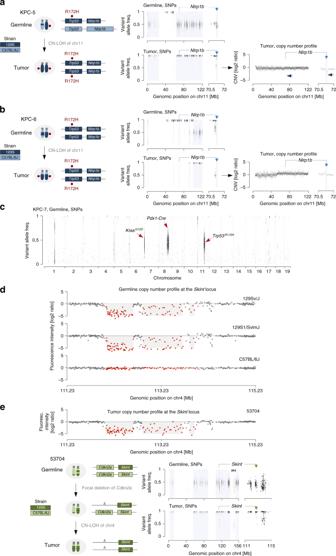Fig. 2: Genetic linkage of strain-specific variants to cancer genes undergoing LOH confound cancer genome analyses. a,bTrp53;Nlrp1haplotype reconstruction by WES-based SNP analysis in germline and tumors of KPC mice (a: KPC-5,b: KPC-6). Genomic regions with heterozygous SNPs contain two distinct alleles: one C57BL/6J- and one 129S-specific haplotype (SNP frequencies: ~0.5; light blue background in SNP-plots). Conversely, regions with SNP frequencies of ~1.0 are pure 129S. Regions without values perfectly match the C57BL/6J reference genome (homozygous C57BL/6J).aIn the germline, heterozygous SNPs confirm presence of two haplotypes: (1)Trp53ENG-129S;Nlrp1129S(engineeredTrp53R172Hallele; strain-specificNlrp1129Svariant) and (2)Trp53WT;Nlrp1C57BL/6J. In the tumor, theTrp53WT;Nlrp1C57BL/6Jhaplotype is lost through CN-LOH (reflecting selective pressure to loseTrp53WT). Homozygosity of theTrp53ENG-129S;Nlrp1129Shaplotype in the tumor manifests as aNlrp1locus deletion when compared to germline (right; CNV plot based on WES withNlrp1locus zoom-in).bIn the germline, theTrp53;Nlrp1haplotype is S129-derived on both copies of chr11. TheNlrp1129Svariant is already homozygous in the germline. CNV analyses relying on tumor/germline comparisons thus fail to detect theNlrp1alteration in the tumor (right; CNV plot based on WES withNlrp1locus zoom-in).cGermline SNP analysis of mouse KPC-7 backcrossed to C57BL/6J for fourteen generations. High SNP densities persist in genomic proximity of engineered alleles.dGermline CNV profiles at theSkintlocus in three inbred mouse strains as compared to C57BL/6J. Red dots, aCGH probes withinSkintlocus alteration (data from ref.6).eUpper panel:Skintlocus CNV profile in primary pancreatic cancer cell culture (compare to germlineSkintalterations in Fig. 2d). Lower panels: WES-basedCdkn2a;Skinthaplotype reconstruction as in Fig. 2a, b. In the germline, heterozygous SNPs confirm presence of two haplotypes: (1)Cdkn2a;SkintC57BL/6Jand (2)Cdkn2a;Skint129S. During tumor evolution, theCdkn2alocus is first somatically deleted (Cdkn2aΔ) on the chromosome carrying theSkint129Svariant (Cdkn2aΔ;Skint129S) followed by CN-LOH of theCdkn2aΔ;Skint129Sallele, reflecting selective pressure to loseCdkn2aWT. Homozygosity ofSkint129Sin the tumor manifests as aSkintlocus deletion when compared to germline (right; CNV plot based on WES withSkintlocus zoom-in). Datasets and data analyses Data and conclusions of this commentary are based on the systematic genetic analysis of our own cohort of over 1000 mouse cancers derived from a variety of distinct mouse models covering different cancer entities. This large cohort of mouse cancers comprise primary cell cultures as well as tissues and was characterized by a series of methods, including array comparative genomic hybridization (aCGH), whole-exome sequencing (WES), long-read sequencing and/or quantitative insertion-site sequencing (QiSeq). Animal experiments, primary mouse pancreatic cancer culture preparation, and maintenance, gDNA isolation were performed as described in detail before [13] , [14] . Genome-wide identification of transposon integration sites in transposon-based mouse models was assessed by using QiSeq and custom bioinformatic analyses as described previously [11] , [15] . Animal studies were ethically approved by the Institutional Animal Care and Use Committees (IACUC) of Technische Universität München, Regierung von Oberbayern and the UK Home Office. Whole-exome sequencing Raw WES data of mouse pancreatic cancers from our cohorts and from Niknafs et al. [1] were analyzed by using a workflow adapted to the analysis of mouse cancer sequencing data which we described elsewhere in detail [14] (source code: https://github.com/roland-rad-lab/MoCaSeq ). In brief, reads were trimmed using Trimmomatic 0.38. BWA-MEM 0.7.17 was used to align reads to the mouse reference genome GRCm38.p6 (with alternate contigs). Picard 2.20.0 and GATK 4.1.0.0 were used for postprocessing (CleanSam, MarkDuplicates, BaseRecalibrator). For LOH analyses from WES data, germline SNP calling was performed with Mutect2 which removes the vast majority of sequencing artifacts. The high number of pseudogenes and segmental duplications in the mouse genome (as compared to the human genome) increases the chance of read mis-mapping. To avoid ambiguous SNP positions resulting from mis-mapping, only reads with a mapping quality of 60 were included in LOH analyses [14] . For CNV detection in mouse and human pancreatic cancers, we used CopywriteR 2.6.1.2 [16] which is based on the analysis of “off-target” reads. “Off-targets” (such as intronic reads), which represent ~20% of all reads in typical WES data sets (due to incomplete removal during standard library preparation), are not affected by variation in capture efficiencies. CopywriteR outperforms algorithms based on the analysis of “on-target” reads (exonic-read based algorithms) for CNV calling from human and mouse WES data [14] , [16] . Array comparative genomic hybridization aCGH data from Niknafs et al. [1] , Maser et al. [2] , Foijer et al. [3] , Foijer et al. [4] , Cutler et al. [6] , Mueller et al. [13] and our own KPC cohort was analyzed using Agilent Genomic Workbench software version 7.0.4.0. Importantly, the identical aCGH array (Agilent, SurePrint G3 Mouse CGH 240 K) was used in all studies, allowing for the direct comparison of strain-specific germline variation at Nlrp1 and Skint loci across all mouse cancer cohorts/genomes. Long-read nanopore sequencing Long-read sequencing libraries were prepared using the Oxford Nanopore LSK109 kit (ONT, Oxford, UK). A total of 400 ng of library was loaded on a promethION flowcell and run for 72 h on a promethION beta sequencer (ONT, Oxford, UK). Base-calling was performed on the promethION compute unit’s GPU using guppy 3.2.8 basecaller. The resulting FASTQ file was mapped to the reference genome GRCm38.p6 using Minimap2 (option map-ont) . Read coverage was extracted using bam-read count ( minimum mapping quality 60 , minimum base quality 5 ). Reporting summary Further information on research design is available in the Nature Research Reporting Summary linked to this article.